The Tissint Martian meteorite as evidence for the largest impact excavation High-pressure minerals in meteorites provide clues for the impact processes that excavated, launched and delivered these samples to Earth. Most Martian meteorites are suggested to have been excavated from 3 to 7 km diameter impact craters. Here we show that the Tissint meteorite, a 2011 meteorite fall, contains virtually all the high-pressure phases (seven minerals and two mineral glasses) that have been reported in isolated occurrences in other Martian meteorites. Particularly, one ringwoodite (75 × 140 μm 2 ) represents the largest grain observed in all Martian samples. Collectively, the ubiquitous high-pressure minerals of unusually large sizes in Tissint indicate that shock metamorphism was widely dispersed in this sample (~25 GPa and ~2,000 °C). Using the size and growth kinetics of the ringwoodite grains, we infer an initial impact crater with ~90 km diameter, with a factor of 2 uncertainty. These energetic conditions imply alteration of any possible low-T minerals in Tissint. The shock-induced, high-pressure phases in Martian meteorites have been used to estimate the dynamics of the impacting bolides and the size of the resulting craters on Mars [1] , [2] , [3] . To date, the high-P phases observed in Martian meteorites include impact-produced glass (maskelynite from plagioclase and pyroxene-composition glass), ringwoodite (γ-polymorph of olivine), akimotoite (ilmenite structure of pyroxene), lingunite (Na-hollandite structure of plagioclase), majorite (garnet structure of pyroxene), tuite (γ-polymorph of merrillite), stishovite (α-TiO 2 structure of quartz) and silicate perovskite (perovskite structure of pyroxene). Most of the high-P phases are polymorphs (more densely packed structure) than the low-P minerals that are listed in brackets above. 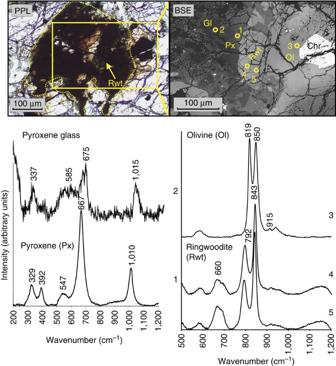Figure 1: A ringwoodite crystal within an impact-melt pocket. The green-coloured ringwoodite (olivine, 75 × 140 μm2) crystal is shown within a large impact-melt pocket (400 × 350 μm2). This crystal is isotropic under cross-polarized light. Selected chemical analyses are listed inTable 1, and more details are given in theSupplementary Information. Raman spectra of this crystal (spot no. 4 and no. 5) show characteristic absorption bands for ringwoodite. The low-P polymorph of olivine nearby displays a different structure (spot no. 3). Numbers next to circles indicate the respective Raman spots. These high-P phases are typically small (<10 μm) and were only observed in isolated occurrences in or near shock-induced melts within the meteorites ( Table 1 ). Tissint was named for a 2011 meteorite fall in Morocco, near the village of Tissint, and was identified to be a Martian meteorite [4] . Being the freshest Martian sample, this meteorite has generated great interest in the community for the possibility of detecting signs of prior Martian life. Table 1 High-P phases (x if present) in Martian meteorites. * Full size table We have conducted a detailed study on eight (8) serial sections from a 10 g piece of this meteorite, which was totally covered by fusion crust. These sections essentially provide a three-dimensional tomography of the sample. After noticing a large ringwoodite grain in a melt pocket, we carefully examined other impact-melt pockets and veins using optical microscopy for texture and mineralogy, electron microprobe (EMP) for chemistry and in situ micro-Raman spectroscopy for definite proof of the structures. Compared with those in the literature data on the structure of similar phases, the chemical and crystal structure information obtained with these coupled methods provide positive identification of the high-P phases (the Supplementary Information ). We observed all nine (9) of the previously identified high-P phases to be present in this single shergottite. The wide occurrence of these high-P phases and their unusually large sizes indicate shock pressures and temperatures of ~25 GPa and >2,000 °C throughout the sample concentrating in the melt pockets. Based on the size and growth rate of ringwoodites, we infer that this sample was excavation and launched from an impact generated by a crater of ~90 km diameter (a factor of 2 uncertainty). This inferred crater size is much larger than that estimated for all other shergottites (3–7 km) (ref. 4 ) to date. Mineralogy The mineralogy and petrography of Tissint resemble other olivine-phyric shergottites (details in the Supplementary Information ) and other pieces of the same fall [5] , [6] . Detailed mineralogy and petrography of Tissint from our study will be reported elsewhere, but a brief summary is given in the Supplementary Information . Shock features Shock features in Tissint are abundant and are suggestive of strong shock metamorphism. All olivines display unusual reddish-brown to black colour imparted by submicron Fe or Fe–O grains formed by shock [7] . Some olivines display undulatory extinction, mosaicism and planar deformation features (PDFs), especially as planar cleavages. PDFs in pyroxenes are clearly visible under crossed-polarized light. Shock-induced glass is also widespread ( Supplementary Fig. S1 ). All plagioclase has been converted to: (a) maskelynite, a diaplectic glass formed by solid-state transformation [8] or (b) glass quenched from shock-induced melting [9] . Thin melt veins of mafic compositions are also present and occasionally emanate from melt pockets ( Supplementary Table S3 ). High-pressure minerals The most distinctive evidence of strong shock is the abundant (2–4 vol. %) melt pockets and their associated high-P minerals ( Table 1 and Supplementary Table S2 ). The sizes of the melt pockets range from 100–350 μm in width and 160–1,000 μm in length. These melt pockets are predominantly associated with olivine grains, residing between the interface of olivine and other minerals. Serial cutting and preparation of thin sections indicate that some melt pockets are interconnected over distances >500 μm. The high-P minerals observed in Tissint include ringwoodite, vitrified perovskite, akimotoite, majorite, lingunite, tuite and stishovite, occurring in different sizes, modes and locations ( Figs 1 , 2 , 3 , Tables 1 and 2 and the Supplementary Information ). An unusually large green-coloured ringwoodite grain (75 × 140 μm 2 ) resides in the edge of a melt pocket ( Fig. 1 ); this is the largest ringwoodite observed in Martian meteorites. Other ringwoodite grains occur as individual smaller grains or thin rims (10–20 μm) along contacts between olivine and the impact-melt pockets ( Supplementary Fig. S4 ), or intergrown with vitrified perovskite in isolated ellipsoidal clasts in a melt pocket ( Fig. 2 ). This is the first report of vitrified perovskite associated with ringwoodite in a Martian sample. The vitrified perovskite also occurs as rims on melt pockets ( Supplementary Figs S4 and S5 ). Figure 1: A ringwoodite crystal within an impact-melt pocket. The green-coloured ringwoodite (olivine, 75 × 140 μm 2 ) crystal is shown within a large impact-melt pocket (400 × 350 μm 2 ). This crystal is isotropic under cross-polarized light. Selected chemical analyses are listed in Table 1 , and more details are given in the Supplementary Information . Raman spectra of this crystal (spot no. 4 and no. 5) show characteristic absorption bands for ringwoodite. The low-P polymorph of olivine nearby displays a different structure (spot no. 3). Numbers next to circles indicate the respective Raman spots. 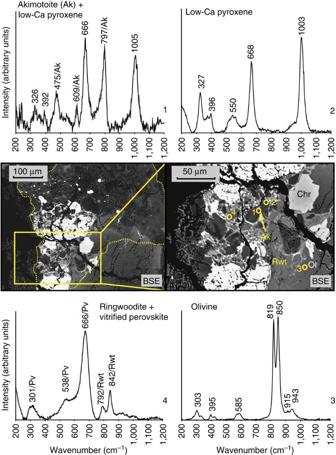Figure 2: High-pressure minerals in the Tissint meteorite. Akimotoite (Ak), ringwoodite (Rwt) and vitrified perovskite in an impact-melt pocket. Ringwoodite was identified in both the centre (no. 4) and rim of the impact-melt pocket. Raman spectra of the low-P equivalents (low-Ca pyroxene and olivine) are shown for comparison (no. 2 and no. 3). Bright minerals within the impact-melt pocket were identified using coupled EMP and Raman spectroscopy as pyrrhotite. Numbers next to the circles indicate the Raman spot analyses. Full size image Figure 2: High-pressure minerals in the Tissint meteorite. Akimotoite (Ak), ringwoodite (Rwt) and vitrified perovskite in an impact-melt pocket. Ringwoodite was identified in both the centre (no. 4) and rim of the impact-melt pocket. Raman spectra of the low-P equivalents (low-Ca pyroxene and olivine) are shown for comparison (no. 2 and no. 3). Bright minerals within the impact-melt pocket were identified using coupled EMP and Raman spectroscopy as pyrrhotite. Numbers next to the circles indicate the Raman spot analyses. 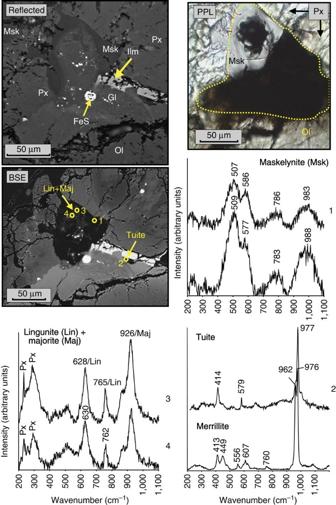Figure 3: Majorite and lingunite in a Martian meteorite. Majorite (Maj), lingunite (Lin) and tuite in an impact-melt pocket. Majorite and lingunite occur in a small plume that originated from the dark impact-melt pocket and intruded into the maskelynite (Msk). For comparison, Raman spectra of these high-P phases were plotted with the low-pressure ones from the groundmass. Numbers next to the circles indicate the Raman analysis spots. Full size image Figure 3: Majorite and lingunite in a Martian meteorite. Majorite (Maj), lingunite (Lin) and tuite in an impact-melt pocket. Majorite and lingunite occur in a small plume that originated from the dark impact-melt pocket and intruded into the maskelynite (Msk). For comparison, Raman spectra of these high-P phases were plotted with the low-pressure ones from the groundmass. Numbers next to the circles indicate the Raman analysis spots. Full size image Table 2 Representative high-P mineral compositions with the related low-P equivalent. Full size table Akimotoite was identified as a small crystal (2–3 μm) replacing the rim of a low-Ca pyroxene fragment ( Fig. 2 ). It is entrained at the centre of a large melt pocket (~530 × 350 μm) in close contact with ringwoodite+vitrified perovskite. Majorite and lingunite (1–2 μm) were observed as polycrystalline aggregates entrained in a plagioclase-glass matrix (maskelynite), surrounded by tiny sulphide droplets ( Fig. 3 ). This is also the first report of majorite and lingunite in a Martian meteorite. Additionally, tuite occurs as minute single crystals (2–3 μm in size; Fig. 3 ) or associated with low-Ca pyroxene in replacement of merrillite ( Supplementary Fig. S5 ). Stishovite is associated with olivine inside a melt pocket ( Supplementary Fig. S6 ). In addition to the high-P minerals, the centre of an impact-melt pocket also contains dendritic crystals (2–3 μm) with a pyroxene-like glass alternating with bright, olivine-like dendrites. The Raman spectra of the regions between the dendrites correspond to a pyroxene-like glass with two predominant broad peaks centred at 664 and 1,011 cm −1 ( Supplementary Fig. S4 ). The diverse array of high-P phases and shock features in Tissint, integrated as a whole assemblage, provides tight and consistent constraints on the P-T conditions of shock metamorphism. The shock features in olivines and pyroxenes (undulatory extinction and mosaicism in olivines, PDF, nano-inclusions in olivines) indicate shock pressures of 26–32 GPa. The presence of shock melts suggests localized temperatures of >1,750 °C. Previously, the formational conditions for maskelynite have been suggested to be a pressure >40 GPa (ref. 10 ). However, more recent studies suggested substantially lower pressures [11] , especially for those formed at higher temperature [12] . Using the method of Fritz et al. , [13] intensity ratios of Raman bands 586–507 cm −1 of maskelynite in Tissint suggest shock pressures between 26 and 40 GPa. The maximum shock pressure and temperature, as constrained by the former perovskite, are 25–40 GPa and 2,000 °C, respectively [14] , [15] , [16] , [17] . Other occurrences of high-P minerals indicate shock pressures of 13–25 GPa and temperatures of 1,700–2,600 °C in melt pockets [17] , [18] , [19] , [20] , [21] , [22] , [23] , [24] , [25] . Furthermore, the absence of lingunite decomposition products (calcium ferrite-type NaAlSiO 4 +stishovite) suggests a P-T upper limit of 24 GPa at ~1,800–2,000 °C (refs 26,27) [26] , [27] . Overall, allowing for the uncertainty in applying available static high-pressure data to Tissint, we derived a peak pressure of ~25 GPa and temperature of ~2,000 °C, with localized shock reaching 40 GPa and 2,000 °C. High-P minerals are formed under the intense pressures and temperatures provided by shock. After their formation, rapid cooling is needed to preserve these phases metastably at low pressure and temperature [11] . Previous studies have estimated the ‘impact duration’, using the size and chemical information of high-P minerals. Beck et al . [2] obtained a shock duration of 10 ms for Zagami, based on diffusion profiles of Cs, Ba and Rb near K-hollandite aggregates; they suggested the crater size to be 1.5–5 km. Other studies [28] , [29] , [30] inferred longer shock durations of seconds to minutes for chondrites from the size of high-P minerals and interface-controlled growth rate [31] . In contrast, however, shock experiments on porous MgO and fused quartz produced 1–3 μm wadsleyite in <1 μs (ref. 32 ). This was used to argue that shock duration is much shorter for wadsleyite that grew from shock-formed melt (growth rate of 1 m s −1 ) (ref. 32 ). It is unclear whether this rapid rate is applicable to ringwoodite, which is a higher pressure polymorph than wadsleyite. In our sections of Tissint, wadsleyite is absent. Thermodynamic data are available only for interface-controlled growth of ringwoodites [30] , [31] . Using the parameters in Mosenfelder et al ., [31] the ringwoodite growth rate is ~2 μm s −1 . Given the observed range, an average size of ringwoodite of 2 μm corresponds to ~1 s. The largest ringwoodite ( Fig. 1 ) cannot be explained by interface-controlled growth, and is likely a result of solid-state transformation or crystallization from shock-formed melt. Therefore, this grain was not used to constrain the shock duration. As the interface-controlled growth is likely more sluggish than solid-state transformation or crystallization from a liquid, the shock durations estimated above may be grossly overestimated. However, the large sizes of ringwoodite in Tissint likely reflect prolonged shock durations. After heating, rapid cooling was achieved in ~50 ms for the centre of the melt pocket and ~20 ms for the rim of the pocket ( Supplementary Fig. S7 ), rendering conditions capable of preserving the high-P minerals observed. Shock durations have been used to infer the burial depth of the original rock within the Martian crust, as well as the impactor size [2] , [33] . The impactor size is estimated using D impactor = τ × v , where τ is the shock duration and v is the impact velocity [2] . Using an average impact velocity of 10 km s −1 on Mars, the impactor size is 10 km. The crater diameter can be approximated using a pi -scaling relation of Melosh [34] , where D proj = τ × ν proj , W is pure kinetic energy, ρ proj is the density of the impactor (3,700 kg m −3 ), ρ target is the density of the basaltic target (2,800 kg m −3 ) and acceleration gravity ( g ) on Mars ( g =3.72 m s −2 ). The crater size resulted by the impactor estimated above is ~90 km. The validity of this estimate depends upon the complex nonlinear process of shock compression and release in the vicinity of a large impact. However, a process has yet to be addressed and modelled using detailed studies with realistic geometries and equations of state. Therefore, this crater-size estimate, conservatively, might be in error by as much as a factor of 2. Shergottites of similar cosmic-ray exposure (CRE) ages have been regarded to be derived from the same source crater [4] . The CRE age of Tissint (0.7±0.3 Myr (ref. 6 ) and 1.10±0.15 Myr (refs 35 , 36 ) is similar to several other olivine-phyric shergottites (for example, EET 79001 NWA 1068, Y 980459 and DaG 476/489, ref. 37 ). Considering the uncertainty, the estimated crater for Tissint is >15 × larger than those suggested for the other shergottites (~3 km) [4] . For those with similar CRE ages, it appears to be contradictory to the previous suggestion. However, none of these shergottites have been thoroughly investigated for their high-P polymorphs. It is more likely that Tissint was launched in the higher-P and higher-T portion of the landing site of the impactor, with other shergottites of the similar CRE age being in proximal less-intense positions of the same crater (ref. 38 ). In such case, the high-P minerals and glasses of Tissint provide a better and more accurate estimation of the crater size as the potential source of the Shergottites. Compared with other Martian meteorites of different CRE ages, the source crater produced shergottites of ~0.7–1.1 Ma CRE age that is possibly the largest. The Tissint meteorite is a unique example of the preservation of a multitude of high-P polymorphs and glasses within a single Martian meteorite. The P-T conditions are tightly constrained from the identified assemblages. However, we feel that the uncertainties encountered in the shock models and the inconsistencies between static and shock experiments, owing to kinetic problems, make sufficient uncertainties in the time dimension. Although the constraints necessary for detailed shock modelling are all present in this meteorite, such a modelling venture is outside the scope of the present study. Notwithstanding, the stronger-than-expected shock metamorphism in Martian meteorites may explain the difficulty in the age dating of shergottites, especially for methods using isotopes of noble gases [39] , [40] . Furthermore, shock metamorphism can easily affect ‘softer materials’ (for example, plagioclase). Given the widely dispersed shock melting observed in Tissint, alteration of other soft minerals (carbonates, halides, sulphates and even organics), especially along grain boundaries, might have occurred. This may in part explain the lack of such minerals in Tissint. Petrography Thin sections were examined using optical microscopy, combined with X-ray maps (Si Kα, Al Kα, Fe Kα and Ca Kα) and the backscattered electron (BSE) images of the sections. The X-ray maps were obtained on a Cameca SX-100 electron microprobe (EMP) at the University of Tennessee. Analytical conditions included an accelerating voltage of 15 keV, a beam current of 20 nA, with 12 μm steps and 75 ms counting times. Modal mineralogy in Tissint was obtained using both BSE and X-ray maps and the image processing software ImageJ. The shades of grey of these maps (0–255) were converted to a histogram, displaying unique peaks corresponding to specific minerals. By selecting a peak (threshold), the amount of a given mineral was measured from a given intensity range of these maps. Using the ImageJ output values, the total area of the specific intensity (a particular mineral) was divided with the total area of the whole section providing the area percentage (vol. %) of a mineral. Errors associated with the measurement of the modal abundances are a function of image resolution and the selection of the threshold values. For confirmation of the results of the above method, we manually contoured the minerals and melt pockets assigning each single phase to a specific colour. EMP analysis Major- and minor-element compositions of minerals and glass were obtained using the Cameca EMP. Olivine, pyroxene and oxide–mineral compositions were measured using accelerating voltages of 15–20 keV, a 20 nA beam current, 1–2 μm beam diameter and counting times of 20 s. Maskelynite, phosphate, sulphide, and glass compositions were determined using a defocused beam with 5 μm size, an accelerating voltage of 10 or 15 keV, with a 10 nA beam current. Detection limits are typically <0.03 wt% for SiO 2 , TiO 2 , Al 2 O 3 , MgO and CaO; <0.04–0.1 wt% for FeO, MnO, Cr 2 O 3 , V 2 O 3 , NiO, Na 2 O, K 2 O and P 2 O 5 . Raman spectroscopy Micro-Raman spectroscopy was conducted on the eight sections of Tissint to verify shock-induced minerals. All Raman spectra were obtained at the Virginia Tech University. The Raman analyses were obtained with a JY Horiba LabRam HR (high resolution) 800 mm spectrometer, coupled with a 514 nm Argon-ion laser and a X100 objective. The laser beam was focused at the surface of the samples with an approximate diameter of 1–2 μm and at ~5 mW laser power. This energy is low enough to avoid appreciable destruction of the sample area. Accumulation times were 30, 60 and 120 s. For each spot analysis, five spectra were acquired and averaged to give the final spectrum. The Raman spectra were corrected by subtracting a baseline, and then peak positions were calculated applying a least-squares curve fitting of combined Gaussian and Lorentzian functions using the LabSpec software provided by Horiba Scientific. Calculation precision was ~±0.2 cm −1 . We examined all melt pockets, melt veins and mineral grains near the melt pockets and veins. Raman spectra of the high-P polymorphs were compared with relevant spectra from open access extensive databases (Handbook of Raman spectra, RRUFF [41] ) and published data. Each high-P polymorph verified by Raman spectroscopy has been coupled with EMP spot analysis for a total mineral identification. How to cite this article: Baziotis, I. P. et al . The Tissint Martian meteorite as evidence for the largest impact excavation. Nat. Commun. 4:1404 doi: 10.1038/ncomms2414 (2013).